Storage of an electric field for photocurrent generation in ferroelectric-functionalized organic devices Organic optoelectronic devices are usually driven by the electric field generated from an electrode potential difference or bias voltage. Although poled ferroelectric domains may produce oriented stray fields, few efforts have been made to utilize them for photocurrent generation in organic devices. Here we show that large net fields caused by incomplete screening during ferroelectric polarization, and which can be ‘restored’ by short voltage pulses, can facilitate exciton dissociation in organic semiconductors. The oriented fields, comparable with that produced by an electrode potential difference (1~10 MV m −1 ), here are found to be responsible for the photocurrent in our devices. A prototype for an organic photodetector driven by such stray fields is demonstrated. The photoresponsivity, without any optimization, can achieve ~0.1 mA W −1 . This study provides a different operation principle for the generation of photocurrent in organic optoelectronic devices. Furthermore, the polarity-tunable photoresponse may lead to new photoresponsive memory devices. Unlike ferromagnetic materials, ferroelectric materials cannot usually exert a stable net field on an object due to screening by free charges or adsorbates from the ambient environment. This significantly limits their potential practical applications. Despite this, much attention has been paid to ferroelectric memory devices [1] , [2] , which are based on the binary conduction states caused by the ferroelectric polarization switching. Recent work [3] indicates that strong electric fields existing at ferroelectric domain walls (2 nm) can separate photo-induced charges in BiFeO 3 (ref. 4 ) with a low internal quantum efficiency (~10%), and the sawtooth-like potential developed inside the device is responsible for an above-band gap photovoltage [5] , [6] , [7] . In contrast, organic optoelectronic devices [8] , [9] , [10] , such as organic photovoltaic (OPV) devices [10] , [11] , [12] , which benefit from light weight, low cost, flexibility and a much higher internal quantum efficiency (close to 100%) [13] , suffer from a strong exciton binding energy. Effective exciton dissociation requires a field of 50–70 MV m −1 (ref. 14 ), which is much larger than that induced by a conventional electrode potential difference (typically 1–10 MV m −1 ). A recent attempt [15] has been made to utilize the ‘strong’ net electric field from poled ferroelectric poly(vinylidene fluoride-trifluoroethylene) (P(VDF-TrFE)) monolayers at electrode interfaces to improve exciton dissociation in OPV devices, despite the fact that the introduction of an organic semiconductor with a low permittivity must induce a large depolarization field ( E d ) [16] , [17] , [18] if there are not enough charges injected for compensation/screening during poling. It was argued that the resultant enhancement originates from chemical reactions at the electrode interfaces that can modify the work function of the electrodes [19] . More recently, OPV devices with unpoled P(VDF-TrFE) as an additive also showed an enhancement of conversion efficiency [14] . Strong local fields were proposed to be responsible for this improvement. However, poled devices did not show additional enhancement. Although the enhancements in ferroelectric functionalized OPV devices were clearly demonstrated, the role of ferroelectric polarization is still not completely understood, and photovoltages are still below the optical gap of the photoabsorber. In addition, whether the net electric field from poled ferroelectric materials, suspended in pure organic semiconductors, can exist stably, and be large enough for exciton dissociation remains unclear. To answer these questions, a better understanding of the physical mechanisms behind ferroelectric induced electric fields in organic semiconductor devices is clearly needed. Here we show that poled ferroelectric domains can produce large oriented net fields inside organic semiconductors with small permittivity for photocurrent generation. Current-voltage characteristics and photocurrent transients [20] , [21] from metal/organic semiconductor/ferroelectric polymer/organic semiconductor/metal (MSFSM) devices were utilized to characterize such fields, which are caused by incomplete compensation of the ferroelectric polarization that undergoes a multi-step polarization process. We note that the average net field, after becoming stable, is comparable with that produced by an electrode potential difference ϕ . A prototype photodetector driven by these oriented stray fields is demonstrated with a photoresponsive memory effect, and a responsivity of ~0.1 mA W −1 under zero bias voltage (passive mode). We also note that even the field induced by ϕ can easily induce ferroelectric polarization, as well as such oriented stray fields, in the devices with nano-scaled ferroelectric components. Such ‘stored’ fields from ferroelectric domains can facilitate exciton dissociation, which is promising for organic optoelectronic devices with multifunction, and the related physics give a deeper insight into the polarization reversal in non-volatile memory devices [17] , [22] , [23] , [24] . Characterization of the devices The multilayer devices were fabricated by similar techniques to those described previously [20] , [21] (see also the Methods section). First, we chose a symmetric MSFSM device structure, with aluminium (Al) as the electrodes, for study to avoid the influence of chemical reactions at each Al/P(VDF-TrFE) interface [19] . Copper phthalocyanine (CuPc) and P(VDF-TrFE) (75/25 mol%) films were chosen as the semiconductor (SL) and ferroelectric layer (FL), respectively. The thickness d f of the FLs is ca . 150 nm. Their molecular structures, as well as the scanning electron microscope image of the multilayer structure, are shown in Fig. 1 . The cross sectional SEM image indicates that the film quality of the FL and SLs in the thicker devices is relatively good. 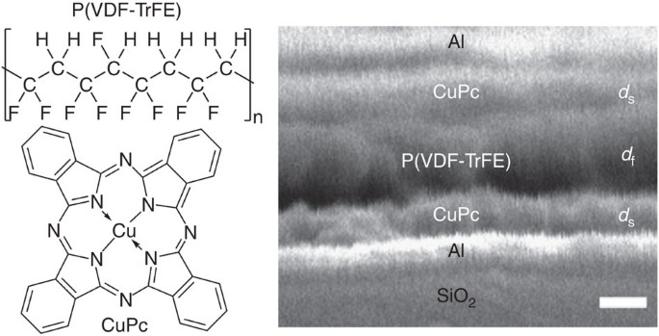Figure 1: Scanning electron microscope image of the MSFSM devices. The scale bar is 100 nm. Thedsanddfare the thicknesses of the CuPc and ferroelectric layers, respectively. The insets are the molecular structure of P(VDF-TrFE) and CuPc. Figure 1: Scanning electron microscope image of the MSFSM devices. The scale bar is 100 nm. The d s and d f are the thicknesses of the CuPc and ferroelectric layers, respectively. The insets are the molecular structure of P(VDF-TrFE) and CuPc. 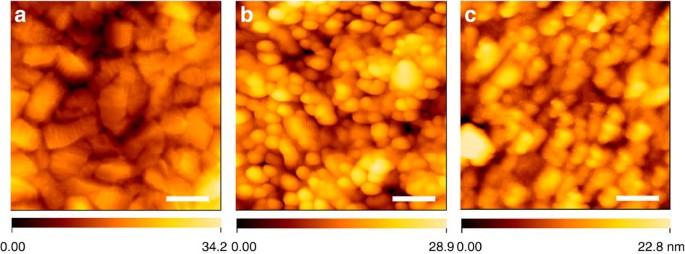Figure 2: Atomic force microscopy images of SL/P(VDF-TrFE)/SL films. (a) The image of the P(VDF-TrFE) film surface, that is,ds=0 nm. (b) The images of the CuPc layers (SL) on the top of P(VDF-TrFE), that is,ds=10 nm and (c)ds=60 nm. The average height for the film withds=0 nm, from valley to top of the film surface, is estimated to be about 9.4 nm. With thedsincreasing, the roughness decreases and the P(VDF-TrFE) particles cannot be distinguished. The scale bars are 100 nm. Full size image Figure 2 shows the atomic force microscopy images of the SL/FL/SL surfaces. For the pure P(VDF-TrFE) film ( Fig. 2a ), the average height, from valley to top of the film surface, is estimated to be about 9.4 nm. The dimensions of the P(VDF-TrFE) grains are ~50–100 nm, which cannot be distinguished in the devices with thicknesses of the SLs d s =60 nm ( Fig. 2c ), indicating a good coverage. We also note that the roughness of the surfaces gradually decreases with increasing d s from 0 to 60 nm. Figure 2: Atomic force microscopy images of SL/P(VDF-TrFE)/SL films. ( a ) The image of the P(VDF-TrFE) film surface, that is, d s =0 nm. ( b ) The images of the CuPc layers (SL) on the top of P(VDF-TrFE), that is, d s =10 nm and ( c ) d s =60 nm. The average height for the film with d s =0 nm, from valley to top of the film surface, is estimated to be about 9.4 nm. With the d s increasing, the roughness decreases and the P(VDF-TrFE) particles cannot be distinguished. The scale bars are 100 nm. Full size image Ferroelectric properties of the devices To confirm the ferroelectric property in our devices with d s =0 (that is, Al/FL/AL structure) and 60 nm, the double-wave method [25] , [26] , [27] , [28] , [29] , [30] was utilized to measure ferroelectric hysteresis loops, which can accurately estimate remnant polarization P r and coercive voltage V c . The detailed procedures are as follows. Current density–voltage ( J – V ) curves were collected with a fast sweep rate ν of 3.7 and 10.6 V s −1 , respectively. The results are shown in Fig. 3a . The J – V curve from the device with d s =60 nm is found to be strongly dependent on the electric poling history ( Supplementary Fig. 1 ). The data (red curve in Fig. 3a ) were collected following many continuous voltage sweeps. For a clear demonstration for both devices, the current amplitude of the thicker device is divided by the rate ratio (10.6/3.7). The small leakage current and dielectric displacement current (see Supplementary Fig. 2 ) have been removed. Both the curves in Fig. 3a exhibit current peaks corresponding to the ferroelectric switching current. The voltages at the peak positions are the V c for these devices. As expected, the device with d s =0 nm (blue curve) demonstrates two symmetric peaks with V c =8.7 V. However, the device with d s =60 nm exhibits six peaks (see peaks 1–6 in the red curve) with the V c at ~10, ~21 and ~28 V, indicating a three-step polarization switching process, in contrast to the two-step process for the MFSM structure [31] . Peaks 1, 3, 4 and 6 can be shown more clearly in the derivative plot of this curve (see Supplementary Fig. 3 ), in which additional peaks combined in peaks 2 and 5 can also be distinguished. Based on P ( V )=∫ JdV / v (refs 27 , 29 ), polarization-voltage ( P – V ) curves are obtained, as shown in Fig. 3b . Typical P – V hysteresis loops can be observed. The Al/FL/Al capacitor exhibits a P r of 8.8 μC cm −2 with a coercive field E c of 58 MV m −1 . The device with d s =60 nm (red curve) exhibits a P r of ~7.5 μC cm −2 . Both values are quite close to the literature data [32] , [33] , [34] . However, compared with the J – V curve, it is difficult to distinguish the ferroelectric switching for peaks 1, 3, 4 and 6 with small amplitudes in the P – V curve. 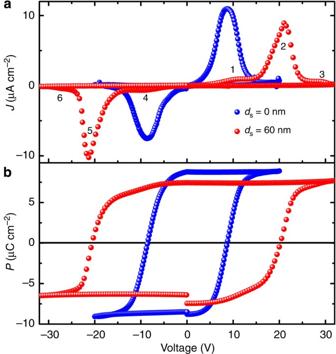Figure 3: Ferroelectric properties of the MSFSM devices. (a) Current density–voltage (J–V) curves for the devices withds=0 (blue) and 60 nm (red). The current peaks are ascribed to the ferroelectric switching. (b) The corresponding polarization–voltage (P–V) hysteresis loops of the devices. Figure 3: Ferroelectric properties of the MSFSM devices. ( a ) Current density–voltage ( J – V ) curves for the devices with d s =0 (blue) and 60 nm (red). The current peaks are ascribed to the ferroelectric switching. ( b ) The corresponding polarization–voltage ( P – V ) hysteresis loops of the devices. Full size image Mechanisms of the multi-peak behaviour Based on the double-layer model with a ferroelectric layer, the fields in the FL ( E f ) and SL ( E s ), without considering the leakage current (which is >1 order smaller than the switching current in our devices), can be expressed as [35] , [36] where ε 0, ε s (=3.6) and ε f (=11) are the dielectric constants of vacuum, CuPc and P(VDF-TrFE), respectively. Therefore, the V c can be expressed as Based on equation (3), we note that the d f deviation (9.4 nm) induced variation of V c is only 0.58 V, which is difficult to be distinguished from the peaks. Therefore, the surface morphology should not be responsible for the split switching current peaks. We note that the V c of peaks 1 ( V c1 ) and 4 are nearly the same as those of the Al/FL/Al capacitor, reflecting that the first term among the three terms in equation (3) is responsible for peaks 1 and 4. The sum of the first and second terms is 19.3 V if we adopt E c =58 MV m −1 and d s =60 nm, thus nearly the same value as that of peak 2 ( V c2 ) or 5, while the P can be estimated to be 0.46 μC cm −2 for peak 3 ( V c3 =28 V) if all the three terms are considered. This value is quite close to the experimental data (~0.31 μC cm −2 ), roughly estimated by integrating peak 3 (1/2 of the integrated values) with indistinguishable edges in Fig. 3b . Since peaks 2 and 5, as well as peaks 1 and 4, are independent of the P , these peaks should originate from either depolarized domains or polarized domains compensated by the charges at the FL/SL interfaces. Considering that no peaks can be observed with a unipolar voltage sweep after poling with the same polarity (see Supplementary Fig. 2 ), the polarization is maintained and the latter mechanism plays the dominant role. Since the p-type SL cannot afford many electrons, most compensating electrons may be directly trapped by the SL. Instead, peak 3 may relate to uncompensated P . Under short-circuit condition ( V =0), E d can by estimated to be ~25 MV m −1 by using equation (1) with P =0.46 μC cm −2 , which is well below the E c , as expected. E s can also be estimated to be ~64 MV m −1 based on equation (2). Based on the above analyses, we now have a clear picture ( Fig. 4 ) for the poled P(VDF-TrFE) domains suspended in organic semiconductors. With a positive V < V c1 , there exist a small amount of carriers, mainly the compensating electrons, in the bottom SL, and there are many holes accumulated at the top FL/SL interface (that is, accumulation state with high carrier density, as denoted by the dark blue colour in Fig. 4 ). The free carriers make the resistance of the two SLs much smaller than that of the FL. Therefore, almost all the V drops across the FL, and the SLs nearly behave as electrodes. The equivalent circuit can be simplified to a capacitor connected with negligible resistors in series, that is, both the SLs act as electrodes. Although each layer can be regarded as an RC element connected in series [37] , where an RC element refers to a parallel resistor–capacitor combination, the capacitive property of the SLs in this case is negligible. When V = V c1 , part of compensated P are reversed (black arrow 1 in Fig. 4 ). 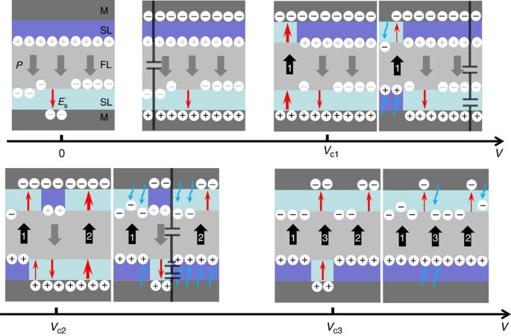Figure 4: Schematic views for the multi-step polarization process. The grey arrows indicate the polarizationPinduced by the previous sweep and the black ones are established in the present sweep. The numbers inside indicate the polarization reversal steps. The grey and black +/− symbols denote positive/negative charges for compensation with the same meaning. Due to the smaller barrier for holes, and the p-type characteristic of the SLs, imbalanced injection occurs just after dipole realignment, as the blue arrows show. This induces uncompensatedPwith electric fieldsEs(red arrows) in the SLs. The line thickness of the red arrows denotes the magnitude of theEs. High carrier density in the SL is depicted by using dark blue, and low carrier density in the SL is demonstrated by using pale blue. Figure 4: Schematic views for the multi-step polarization process. The grey arrows indicate the polarization P induced by the previous sweep and the black ones are established in the present sweep. The numbers inside indicate the polarization reversal steps. The grey and black +/− symbols denote positive/negative charges for compensation with the same meaning. Due to the smaller barrier for holes, and the p-type characteristic of the SLs, imbalanced injection occurs just after dipole realignment, as the blue arrows show. This induces uncompensated P with electric fields E s (red arrows) in the SLs. The line thickness of the red arrows denotes the magnitude of the E s . High carrier density in the SL is depicted by using dark blue, and low carrier density in the SL is demonstrated by using pale blue. Full size image Since V c2 can be determined from equation (3) ( P =0), which is based on the double-layer model (that is, two capacitors in series) with d s =60 nm, the FL and one of the SLs should show a capacitive behaviour. This is reasonable since the small amount of free carriers in the bottom SL are not enough for a full polarization, and such carriers will be consumed (low carrier density is denoted by a pale blue colour in Fig. 4 ) after peak 1, and the resistance of the remaining part of the bottom SL becomes very large (as a capacitor that can share a part of the V ), leading to E f < E c . Only when V = V c2 ( E f = E c ), the related P can be reversed (black arrow 2). It should be pointed out that the E s (see the red arrows in Fig. 4 ) in the SLs just after dipole realignment ( E f = E c ) is very large before compensation. By integrating peaks 1 and 2 in Fig. 3b , the related P can be estimated to be ~0.84 and ~6.4 μC cm −2 , respectively. Based on equation (2), the corresponding E s with d s =120 nm (that is, the top SL is also partially depleted) just after dipole realignment can be calculated to be 136 and 707 MV m −1 , which are much larger than the values just before realignment, that is, 51 and 124 MV m −1 , respectively. The E s can be amplified [35] by dipole alignment without being compensated. Even without ferroelectric polarization, the latter values are still much larger than those in pure CuPc devices with the same thickness (270 nm), that is, 37 and 78 MV m −1 , respectively. Obviously, the E s just after dipole realignment can be large enough to induce charge injection through tunnelling effects or thermionic emission, and even lead to breakdown of the SL (the breakdown field of ITO/CuPc/Al devices is found to be ~250 MV m −1 by using a reverse bias sweep), generating enough charges at the SL/FL interfaces for compensation with a much decreased E s , though both contacts in the devices are blocking type (as the schematic view shows in the inset of Supplementary Fig. 1 ) with a smaller barrier for holes. Such massive charge generation at the SL/FL interfaces can be responsible for the stably maintained P with relatively good compensation. When V = V c3 ( V c of peak 3), the E s from uncompensated P produced by the previous cycle in the bottom SL is overcome, and realignment occurs for the related dipoles (black arrow 3). In this case, the device can be regarded as two capacitors and one voltage source connected in series. For all the steps just after dipole realignment, imbalanced injection (see the blue arrows), due to a smaller hole-injection barrier and the p-type characteristic of the SLs, can lead to uncompensated P , which immediately induces an E s in the top SL with E d < E c , and most holes will accumulate in the bottom SL. Following this, a negative sweep process produces an opposite behaviour. It is worth mentioning that there are ranges for the highest occupied molecular orbitals and lowest unoccupied molecular orbitals of the SLs in literatures. Therefore, easier electron injection, with a smaller barrier, is also possible in reality. However, the poor electron accommodation in the SLs still cannot support many injected electrons, and most of these will be trapped by the FL, similar to the above situation with the same directions of E s . Therefore, such imbalanced injection can still produce the same behaviour, although the charge distribution would be different. Based on the above-mentioned multi-step polarization reversal process, we can develop a schematic view of the charge, potential and electric field distribution inside the devices just after poling (for example, the device is poled with a V > V c3 as shown in Fig. 5 ). The small Debye screening length of the electrodes [38] and dielectric polarization inside the SLs are not considered. For the poled MSFSM device with P r in the short-circuit condition, one of the SLs is in the accumulation mode, with the compensating charge of + q distributed as the red area in the right SL of Fig. 5a . The screening length L D = determines the width of the accumulation layer, which is usually less than 5–20 nm (refs 2 , 39 ) for organic semiconductors, where k , T , e and n are the Boltzmann constant, absolute temperature, the charge of an electron and carrier density, respectively. However, the charge distribution in the left side is quite different. In addition to the injected electrons during poling, the E d (< E c ) may also induce electrons in the electrode, and the total charges at the surfaces of the left SL will be − q (blue areas). The induced potential drop in the SLs after poling produces the E d as well as E s , as the grey arrows depict in Fig. 5b . Since the SLs are not ideal insulators, electrons can continue to be injected due to the E s until the drift current I dr finally equals the diffusion current I di with an opposite polarity (see the red arrows). The corresponding L D will be determined by the acceptor density in the SL, as well as at the surface of the FL. Within the range of L D , the SL is not neutral, and there is still a built-in field with bent band. Both the stray fields from uncompensated and compensated P by the charges in the SLs can be utilized. However, no fields can ultimately be generated in the SLs if all the compensating charges are directly trapped by the FL. 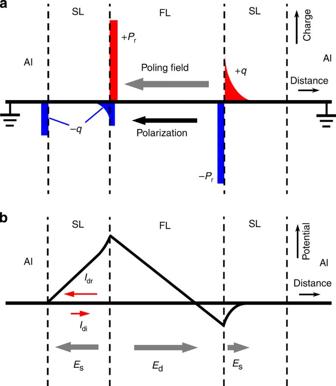Figure 5: Schematic views for the MSFSM devices after poling. (a) Charge distribution after poling. FL, ±qand ±Prare the P(VDF-TrFE) layer, compensating and the polarization charges, respectively. (b) The electrostatic potential profile and the relevant electric fields in the SL (Es) after poling, as well as the depolarization field (Ed). TheEsin the left side just after poling becomes stable only when the induced drift current (Idr) equals the diffusion current (Idi). Under short circuit conditions, the simplest sawtooth-like potential may contribute to the photocurrent in the MSFSM devices. Figure 5: Schematic views for the MSFSM devices after poling. ( a ) Charge distribution after poling. FL, ± q and ± P r are the P(VDF-TrFE) layer, compensating and the polarization charges, respectively. ( b ) The electrostatic potential profile and the relevant electric fields in the SL ( E s ) after poling, as well as the depolarization field ( E d ). The E s in the left side just after poling becomes stable only when the induced drift current ( I dr ) equals the diffusion current ( I di ). Under short circuit conditions, the simplest sawtooth-like potential may contribute to the photocurrent in the MSFSM devices. Full size image Photoresponse of symmetric MSFSM devices To verify the ‘stored’ E s after poling, and its effect upon exciton dissociation, the photoresponse of the symmetric MSFSM devices with d s =60 nm was examined, since photogenerated excitons in the SLs are a good ‘sensor’ for electric fields, as shown in Fig. 6 . Before poling, only a small current transient (the dark lines in Fig. 6 ) is detected, which could be ascribed to interfacial effects (such as a dipole layer effect), pyroelectric or self-poling effect. After poling at −30 ( Fig. 6a ) and +30 V ( Fig. 6b ), large photocurrent transients ( J tr ), consisting of an ON-state ( J on ) and an OFF-state transient upon light on and off, with positive/negative directions, are detected for these devices. The positive J tr is caused by a light-induced charging process, while the negative J tr originates from the discharging or recovery process [20] . As can be seen, the polarities of the J tr induced by positive and negative poling are opposite to each other. The initial states after poling are not stable, and the large J tr decays into a stable value (~1/6 of the initial value) after ~6.5 h. By integrating the stable J on , the extracted charges Q from the device can be estimated to be ~10 −4 μC cm −2 , which is 3–5 orders smaller than the polarization charge density at E c . Therefore, the photogenerated charges cannot induce a back-switching process in the FL. We note that quantum processes play a dominant role since the photoinduced pyroelectric current is found to be <0.20 μA cm −2 (see Supplementary Figs 4 and 5 ) with a temperature change of 0.15 K, and an opposite polarity, which can be predicted from the release of compensation charges upon the photoinduced heating process. In addition, the small photoinduced pyroelectric current is quite stable. Even a weak effective intensity of ~15 μW cm −2 can also induce a similar behaviour without the contribution of the pyroelectric current (see Supplementary Fig. 6 ). 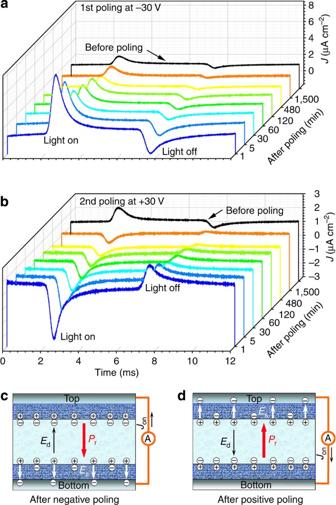Figure 6: Photoresponsive memory effect. Photoelectric memory effect from the MSFSM devices withds=60 nm, poled at −30 V (a) and +30 V (b). The resultant unstable photocurrent transients gradually decay into a stable state after 6.5 h, which are induced by the stray field from the poled FLs. The polarity-tunable behaviour can be observed from all the samples (>10). (c) and (d) show the schematic diagrams for the electric field distribution after poling at negative and positive voltages, respectively. The polarity of the ON-state (Jon) transients upon light on matches well with the predictions from the direction of the remnant polarization (Pr), that is, thePrdirection is always consistent with that ofEsorJon. Figure 6: Photoresponsive memory effect. Photoelectric memory effect from the MSFSM devices with d s =60 nm, poled at −30 V (a) and +30 V ( b ). The resultant unstable photocurrent transients gradually decay into a stable state after 6.5 h, which are induced by the stray field from the poled FLs. The polarity-tunable behaviour can be observed from all the samples (>10). ( c ) and ( d ) show the schematic diagrams for the electric field distribution after poling at negative and positive voltages, respectively. The polarity of the ON-state ( J on ) transients upon light on matches well with the predictions from the direction of the remnant polarization ( P r ), that is, the P r direction is always consistent with that of E s or J on . Full size image Based on the current polarities, the electric field directions inside the devices just after negative and positive poling are as in Fig. 6c,d , respectively. The J on direction after negative poling goes from the bottom to top electrode in the external circuit (see the arrow in the external circuit of Fig. 6c ). Similarly, positive poling induces a J on1 with an opposite polarity, as shown in Fig. 6d . These match well with the prediction from the ferroelectric polarization switching, that is, the polarization direction is consistent with that of E s (the E s in the narrow accumulation layer is not depicted). It is noted that the bi-state photoresponse can be repeatedly switched by positive and negative poling, indicating that no significant decomposition occurs in the SLs. Such behaviour can also be clearly observed in other devices with d s ≥30 nm, even poled by an ultra-short pulse of ~1 ms. Their stable signals can be temporarily suppressed by applying a small bias voltage (<1 V) during the photocurrent measurements. For instance, Supplementary Fig. 7 demonstrates the Q –| V | curve from the device with d s =150 nm, in which Q is obtained by integrating the J on . The value of Q equals zero when V =0.8 V. Based on equation (2), the effective average field in the SLs can be calculated to be approximately 4.0 MV m −1 , comparable with the field caused by ϕ . Considering the pyroelectric contribution and band bending at the SL/FL interfaces, the E s would be larger. The slow decay process can be ascribed to the imprint effect [27] , [40] that is, free or compensating charges in the SLs are gradually injected and trapped by the FL for a better compensation due to the E d . Photoresponse of asymmetric MSFSM devices We also investigated asymmetric devices with a structure of ITO/CuPc/P(VDF-TrFE)/fullerene (C 60 )/Al ( d s =50 nm), which can exhibit a similar poling effect. The inset of Fig. 7a is the related energy level alignment for this structure. Since the device with d f =150 nm can hardly exhibit the stable polarity-tunable photoresponse due to a large contribution of ϕ , the devices with d f =900 nm were studied. In this case, the average field caused by ϕ in the devices is dramatically decreased. The tunable behaviour with a large photoresponsivity from the device is demonstrated as in Fig. 7 . Before poling, the device exhibits a positive J on (black curve) as expected (that is, holes move from ITO to the Al electrode). After poling at −90 V ( Fig. 7a ), the J on decreases into a slightly smaller value within 1 min and nearly becomes stable. Considering that poling can cause massive charge injection on both sides, in spite of the nominated depletion states, band bending at the SL/FL interfaces may kill the electric field from ϕ in the bulk region of the SLs. Although the E s in the accumulation layers can produce photocurrent, this cannot compensate the decrease of the photocurrent contributed from ϕ . Especially, most injected charges may be directly trapped by the FL, which cannot contribute to photocurrent generation. 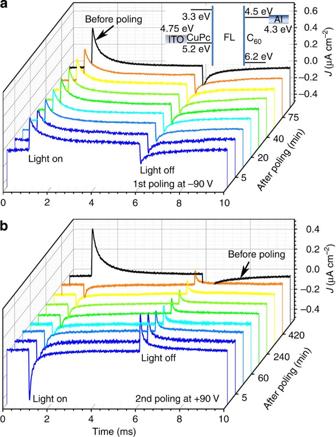Figure 7: Photoresponses from poled thick asymmetric devices. (a) Photocurrent transients after poling at −90 V, which are slightly decreased, compared with those before poling. The response does not show further decay. The inset is the schematic view of the energy levels in the asymmetric ITO/CuPc/FL/fullerene (C60)/Al devices. (b) Photocurrent transients with opposite polarity after poling at +90 V. The response gradually decreases into a stable signal after nearly 2 h, due to the fields in the accumulation layer of the SL. Even without the stray fields from the uncompensatedP, the photoresponse can still achieve 0.1 mA W−1. Figure 7: Photoresponses from poled thick asymmetric devices. ( a ) Photocurrent transients after poling at −90 V, which are slightly decreased, compared with those before poling. The response does not show further decay. The inset is the schematic view of the energy levels in the asymmetric ITO/CuPc/FL/fullerene (C 60 )/Al devices. ( b ) Photocurrent transients with opposite polarity after poling at +90 V. The response gradually decreases into a stable signal after nearly 2 h, due to the fields in the accumulation layer of the SL. Even without the stray fields from the uncompensated P , the photoresponse can still achieve 0.1 mA W −1 . Full size image It is notable that an opposite J on can be detected after poling at +90 V with a large responsivity of ~0.23 mA W −1 . After 2 h, the response becomes stable, with a responsivity of ~0.1 mA W −1 , almost 1/2 of the initial value. In spite of the small barrier at the ITO/SL interface, which can be overcome by thermal energy, both the SLs are in the accumulation state after positive poling. As a result, only one peak can be observed in the positive J – V curve (see the Supplementary Fig. 8 ), that is, there are no barriers for charge injection in this case. The J tr , partly cancelled by the pyroelectric effect and ϕ , should be produced by the E s in the narrow accumulation layers of the SLs. It is natural that the J on decays much faster since there is no screening or imprint process for uncompensated P , which exists in the above symmetric devices. The J tr due to the ferroelectric property under passive mode ( V =0 V), that is., without consuming energy during operation, is quite applicable. Although it is 1–3 orders smaller than those of the most-advanced organic photodetectors [8] , there is significant scope for improvement, such as by decreasing ϕ , or adopting different SLs (for example, bulk-heterojuction SLs). It is notable that the device capacitance is only 0.56 nF at 1 Hz. Instead, the capacitance of the ITO/CuPc (50 nm) per Al cell with a similar responsivity (see the Supplementary Fig. 9 ) is very large (2.9 nF). Since the stray field from the FL is independent of thickness, unlike the field caused by ϕ , this new operation principle would be suitable for high-speed operation by increasing d f to decrease the RC constant. In addition, the appearances of the OFF-state transients and small dark current make the signal inherently more detectable. Although the memory devices with binary conduction states, caused by the depletion/accumulation of compensation charges for ferroelectric polarization, has been intensely studied, we have now shown that the E s from uncompensated P , the oriented local E s in the accumulation layers and the amplified E s with ϕ due to linear dielectric property is also very promising, especially for optoelectronic devices. All of these, as well as the random distributed local field [14] , can play significant roles in the device operating in transient mode. Unlike the field caused by ϕ , the oriented local E s is independent of d f , and even thick devices with small capacitance can also show significant photoresponse. This architecture would be suitable for high-speed operation. Larger E s could be obtained if the field from ϕ is small enough. In addition, blocking contacts are preferred for the E s from uncompensated P . Since the polarity of transient photocurrent can be tuned, it may lead to a new optoelectronic device with memory function. The oriented local E s would also contribute to photocurrent generation in conventional dc devices. Considering that the SLs with free carriers inside can act as electrodes for poling, only the dimension of such SLs determines the V c (= E c d f ). The ϕ in dc devices with small dimensional ferroelectric components, such as the OPV devices in previous reports [14] , [15] , may be sufficient for poling. As shown in Supplementary Note 1 and Supplementary Fig. 10 , the ITO/CuPc/FL/CuPc/Al devices with an ultrathin FL exhibit a very small V c comparable with ϕ . Related current peaks can even cover the zero bias voltage, which may reflect a partial self-poling process. Compared with the devices without the FLs, the device show significantly enhanced photovoltaic performance. However, it is difficult to determine the contribution from the oriented E s , since random distributed local fields and field amplification due to its linear dielectric property may also help for photocurrent generation. Considering an even smaller dimension of the ferroelectric components and a larger ϕ with two injecting contacts (the resultant bipolar injection can induce plenty of free carriers for poling) of the OPV devices in the previous reports [14] , [15] , the ferroelectric polarization may have already occurred, and the resultant oriented E s may play a partial role for the performance enhancements in their devices. Since the large amount of free charges due to the dc photocurrent, which may induce good compensation for polarization, there should not be a large E s across the whole devices, as proposed in Yuan et al. [15] In summary, the double-wave method and photocurrent transients have been employed to probe net fields in organic materials from poled P(VDF-TrFE) films. It has here been directly demonstrated that the oriented net field related to ferroelectric polarization can facilitate exciton dissociation in organic semiconductors. The surface potential at the interface of the ferroelectric components can provide a stable field comparable with that produced by an electrode potential difference. This gives a hint to an artificial ‘sawtooth potential’ by using a combination of ferroelectric layers and semiconductor layers with a low permittivity. A novel operation principle for organic photodetectors is demonstrated by using a prototype device driven by the stored stray fields from ferroelectric dipoles, which exhibits a stable responsivity of 0.1 mA W −1 . The polarity-tunable photoresponse lends itself to application as a multifunctional memory device. Such stray fields may also play an important role for the photocurrent generation in OPV devices. Combined with the other advantages of ferroelectric materials, such as a field amplification effect [35] , [41] and the capability for surface modification of electrodes [19] , organic devices functionalized by ferroelectric materials are quite promising for optoelectronic devices [8] even with memory functionality. Device fabrication All the materials in this work are commercially available and were used as received. Substrates were pretreated by sequential ultrasonication with 2-propanol, acetone and chloroform for 15 min each. In addition to the ultrasonication, the patterned ITO substrates were then treated with ultraviolet-ozone for 2 min, which is known to raise its work function [42] . After the deposition of the CuPc films at a pressure of 5 × 10 −4 Pa with a rate of 0.05 nm s −1 by using vacuum vapour deposition, the P(VDF-TrFE) layers were fabricated via spin coating from 40 mg ml −1 (for thick films) and 2 mg ml −1 (for the ultrathin films) dimethylformamide (DMF) solutions. The films were annealed in a vacuum at 145 °C for 60 min. The top SLs and aluminium (Al) electrodes were then thermally evaporated without further annealing. Film thickness was determined by a Dektak 150 surface profilometer. The effective area for each device is 0.04 cm 2 . All the measurements were carried out in a vacuum at room temperature. Morphology characterization The cross sectional SEM image was recorded by a Hitachi S-4300 field emission scanning electron microscope in secondary electron mode. The atomic force microscopy images were collected by an atomic force microscope (Seiko II, SPA-300HV). Electrical measurements Samples were fixed in a home-made vacuum chamber with a quartz window and illuminated from the bottom electrodes, which are defined as the positive electrodes. The two electrodes of the samples were connected to a current amplifier (Keithley 428). Amplified voltage signals were then recorded by an oscilloscope (Tektronix TDS5104B). Current values were calculated based on the gain of the amplifier and the recorded voltage signals. A green laser (532 nm) modulated by a chopper was adopted as the light source for the symmetric devices. A poling voltage pulse (> V c ) of 5 s was utilized. Taking into account the transmittance of the bottom Al electrode (~5%), the effective incident laser intensity was adjusted to ~100 mW cm −2 . For the thick asymmetric devices, a yellow (~590 nm) light-emitting diode modulated by a function generator (Tektronix AFG320) with a home-made driving circuit was utilized. Light intensity was fixed at ~2 mW cm −2 . Photoresponsivity was calculated by dividing the peak values of J on by the incident light intensity. All the J–V curves were collected by a dc voltage current source (ADCMT 6241A) under dark conditions. Device capacitances were recorded by an LCR metre (ZM2375, NF Corporation) with a probing signal of 100 mV. How to cite this article : Hu, L. et al. Storage of an electric field for photocurrent generation in ferroelectric-functionalized organic devices. Nat. Commun. 5:3279 doi: 10.1038/ncomms4279 (2014).